Comments on identifying causal relationships in nonlinear dynamical systems via empirical mode decomposition 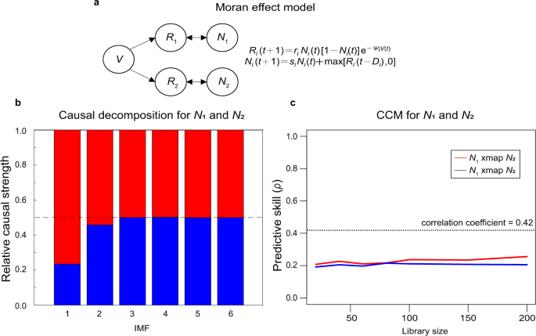Fig. 1: Causal decomposition fails to falsify spurious causations presented in Moran effect model. aMoran effect model is a 5-variate difference equation model in which variablesN1andN2have no causal relationship, but have a significant correlation in their time series due to shared external forcing,V. We ran this model for 10,000 time steps with the parameter set [r1= 3.4,r2= 2.9,ψ1= 0.5,ψ2= 0.6,s1= 0.4,s2= 0.35,D1= 3,D2= 3,R1(0) =R2(0) = 1,N1(0) =N2(0) = 0.5], but retaining only the last 200 steps for analysis. Because of the strong correlation betweenN1andN2.bThe causal decomposition method, incorrectly concluded causation according to IMF 1 and 2, even thoughN1andN2do not interact. Here, causal decomposition is performed under 1000 ensemble EMD with noise levelr= 0.085 selected based on the criteria of maximizing the separability but maintaining orthogonality of the IMFs, following the Matlab codes provided in Yang et al.1. In contrast,cCCM had no convergence (i.e., no improvement in CCM skill with increasing library size) in cross-mapping betweenN1andN2, and thus correctly concluded no causation betweenN1andN2. 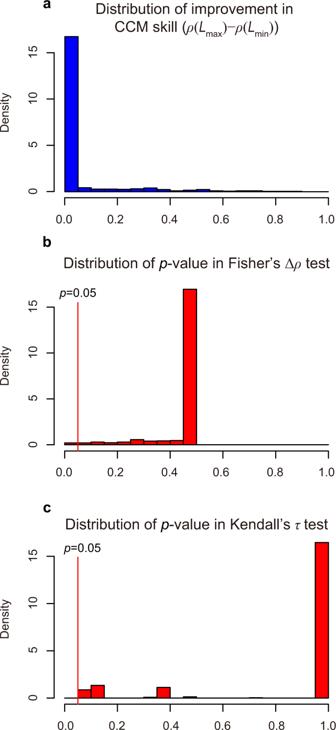Fig. 2: CCM analysis for paired white noises. White noise time series were generated from 10,000 simulations and all time series were trimmed to length = 10, following Yang et al.1. In total, we performed CCM analyses between 1000 random pairs of white noises. To evaluate convergence of CCM, we calculated three indices:aimprovement in CCM skill from minimal (L= 2) to maximal library length (L= 10);bpvalue for testing the significance of the improvement in CCM skill using Fisher’s ΔρZ test; andcpvalue for testing the significance of monotonic increasing trend in CCM skill using Kendall’sτtest. In a majority of cases, improvements in CCM skill were very small and close to zero, indicating no convergence (a). As such, false positives in both Fisher’s Z test (b) and Kendall’sτtest (p< 0.05) (c) occurred, with very low probability. In summary, the probability of detecting spurious causation in paired short white noise was very low; this was opposite to conclusions of Yang et al.1based on the incorrect definition of CCM. Further information on research design is available in the Nature Research Reporting Summary linked to this article.